Programmed folding of DNA origami structures through single-molecule force control Despite the recent development in the design of DNA origami, its folding yet relies on thermal or chemical annealing methods. We here demonstrate mechanical folding of the DNA origami structure via a pathway that has not been accessible to thermal annealing. Using magnetic tweezers, we stretch a single scaffold DNA with mechanical tension to remove its secondary structures, followed by base pairing of the stretched DNA with staple strands. When the force is subsequently quenched, folding of the DNA nanostructure is completed through displacement between the bound staple strands. Each process in the mechanical folding is well defined and free from kinetic traps, enabling us to complete folding within 10 min. We also demonstrate parallel folding of DNA nanostructures through multiplexed manipulation of the scaffold DNAs. Our results suggest a path towards programmability of the folding pathway of DNA nanostructures. DNA is an attractive material for building nanostructures because of its programmability, stability and the feasibility of mass production [1] . The DNA origami technique provides a platform to design DNA-based nanostructures with site-specific modifications at one nucleotide resolution [2] , [3] , [4] , [5] , [6] , [7] , [8] , [9] , [10] . In the DNA origami technique, a long single-stranded DNA (the scaffold DNA) makes base pairing with short oligonucleotides called staple strands. Each staple strand has multiple binding sites, thereby bringing together otherwise distant parts of the scaffold DNA (that is, cross-over points), which in turn induces folding of the scaffold DNA into a designed nanostructure [2] . Unlike protein and RNA molecules, whose folding landscapes are evolutionarily tailored [11] , [12] , [13] , [14] , [15] , DNA origami structures typically navigate a much more rugged and complex folding landscape with many kinetic traps. Most notably, owing to existence of random complementary bases, a single-stranded scaffold DNA has numerous internal structures at both secondary and tertiary structure levels, which prevent binding of the staple strands and hamper the folding process. Thermal annealing is thus the most widely used method for DNA origami folding, in which internal structures of the scaffold DNA are removed at a denaturing temperature of 80 °C. The scaffold DNA, mixed with its staple strands, is slowly cooled to reach the designed structure with the minimum energy configuration. This thermal annealing method has been able to successfully fold various DNA origami structures, even including three-dimensional structures [3] . In addition, it was recently reported that by maintaining the annealing process at a constant temperature, the rate of thermal folding can be dramatically increased, completing the entire folding process within only tens of minutes [16] . However, the annealing method, including constant temperature incubation, is an inherently one-pot reaction, meaning that all the constituting molecules are allowed to react and fold at the same time. It is difficult to separate individual elementary processes and gain insights towards the role of each process in the folding of DNA nanostructures. In this work, we demonstrate that the single-molecule force spectroscopy [17] , [18] , [19] , [20] , [21] , [22] enables dissection of the self-assembly process of DNA origami structures. Through modulation of the energy landscape of selected single molecules [23] , [24] , [25] , [26] , [27] , [28] , folding of DNA nanostructures can be decomposed into three molecular processes: mechanical stretching of the scaffold DNA, its base pairing with the staple strands and displacement between the bound staple strands. Our mechanical folding method sheds light on the folding mechanism of DNA nanostructures, suggesting a path towards a capability to design and modulate the folding pathway of DNA origami. Mechanical folding pathway of DNA origami We propose a folding pathway for DNA nanostructures, in which the energy landscape of the scaffold DNA is selectively modulated with the single-molecule force spectroscopy ( Fig. 1a ). Through internal base pairing, the scaffold DNA contains many secondary structures ( Fig. 1a , state I). In thermal folding protocols, these secondary structures are removed by heating the scaffold DNA. An alternative way to remove such internal structures is to mechanically stretch the single-stranded scaffold DNA with single-molecule force methods [29] . One crucial difference from thermal denaturation is that selective melting of the scaffold DNA is performed essentially at room temperature or 36 °C. Thus, the scaffold DNA can be hybridized by simply introducing the staple strands ( Fig. 1a , state II), which prevents formation of internal structures in the scaffold DNA even when the mechanical tension is removed. 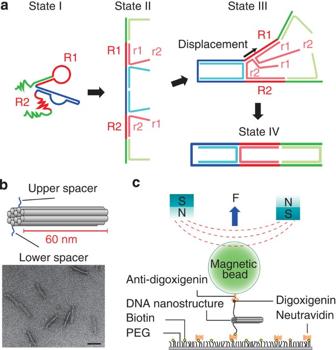Figure 1: Schematic for DNA nanostructure folding with magnetic tweezers. (a) Design of the folding pathway. In the absence of external tension, the scaffold DNA is in state I due to the formation of secondary structures. After denaturing this secondary structure with force, hybridization of staple strands yields state II. In state II, staple strands with same sequence (marked with the same colour) are redundantly bound to one scaffold DNA, because each staple strand has multiple binding sites for scaffold DNA. The nanostructure is folded by removing redundant staple strands with strand-displacement reactions, forming cross-over points. State III shows an intermediate state during the folding process; one blue staple strand has already been displaced, while a red staple strand is being removed from the region R1. After redundant staple strands are removed, the folding is completed (state IV). (b) Designed shape of a DNA nanostructure with ten helices (upper) and electron microscopy image of thermally annealed DNA nanostructures (lower). Scale bar, 50 nm. (c) Schematic of a DNA nanostructure folding experiment using magnetic tweezers. A long, single-stranded scaffold DNA is immobilized onto a PEG-coated slide by biotin–neutravidin interaction, with a magnetic bead attached to the other end of the scaffold DNA via digoxigenin-anti digoxigenin. Figure 1: Schematic for DNA nanostructure folding with magnetic tweezers. ( a ) Design of the folding pathway. In the absence of external tension, the scaffold DNA is in state I due to the formation of secondary structures. After denaturing this secondary structure with force, hybridization of staple strands yields state II. In state II, staple strands with same sequence (marked with the same colour) are redundantly bound to one scaffold DNA, because each staple strand has multiple binding sites for scaffold DNA. The nanostructure is folded by removing redundant staple strands with strand-displacement reactions, forming cross-over points. State III shows an intermediate state during the folding process; one blue staple strand has already been displaced, while a red staple strand is being removed from the region R1. After redundant staple strands are removed, the folding is completed (state IV). ( b ) Designed shape of a DNA nanostructure with ten helices (upper) and electron microscopy image of thermally annealed DNA nanostructures (lower). Scale bar, 50 nm. ( c ) Schematic of a DNA nanostructure folding experiment using magnetic tweezers. A long, single-stranded scaffold DNA is immobilized onto a PEG-coated slide by biotin–neutravidin interaction, with a magnetic bead attached to the other end of the scaffold DNA via digoxigenin-anti digoxigenin. Full size image From the state II, folding of the DNA nanostructure is completed mainly through one type of process—displacement among the bound staple strands. In the DNA origami structure, each staple strand is designed to bind multiple regions on the scaffold DNA, thereby holding those regions together with a well-defined geometry. Thus, in the state II, multiple staple strands with the same sequence bind different binding regions of the scaffold DNA (see Fig. 1a for the staple strands with the same colour). Displacement between these same staple strands can be initiated by simply quenching the mechanical tension on the scaffold DNA. On release of mechanical tension, the configurations of scaffold DNA in state II rapidly collapses to those in state III ( Fig. 1a ). In the state III, the staple strands of the same sequence compete for the identical binding site in the scaffold DNA, which results in displacing one of the two staple strands. Such DNA displacement process is shown to be highly cooperative [30] , favouring efficient kicking out of one staple by the other rather than stagnant tug-of-war between the staple strands. When all the redundant staple strands are released, folding of the DNA nanostructure is completed ( Fig. 1a , state IV). Real-time observation of folding of a DNA origami structure To demonstrate the folding pathway of DNA nanostructures contemplated above, we designed a DNA origami structure, a honeycomb lattice with ten helices, made of a scaffold DNA with 1,899 nucleotides and 51 staple strands ( Fig. 1b , Supplementary Fig. 1 and Supplementary Table 1 ). Figure 1b shows an electron microscope image of the folded helix bundles induced by conventional thermal annealing. To selectively denature the scaffold DNA at room temperature, we selected magnetic tweezers as a tool for the single-molecule force spectroscopy [17] , [18] ( Fig. 1c ). Magnetic tweezers can manipulate single DNA molecules with pico-newton force while probing their end-to-end distances with a nanometre resolution [17] , [18] , [19] , [20] , [26] , [31] , [32] , [33] , [34] , [35] , [36] . In addition, different from other methods for single-molecule force spectroscopy, magnetic tweezers inherently permits multiplexed manipulation, which allows us to fold DNA nanostructures in a highly parallel manner in one experiment (see below). We immobilized a single scaffold DNA onto a polyethylene glycol (PEG)-coated glass surface and monitored its extension during the folding process ( Figs 1c and 2a , and Supplementary Fig. 2 ). In the absence of applied force, extension of the single-stranded scaffold DNA was close to zero ( Fig. 2a , state I-a). The folding was initiated by stretching the scaffold DNA with force, which was to remove the internal structures and expose binding sites for the staple strands. However, the extension was shorter than that of the fully stretched state, because some of the internal structures persisted even at 5 pN ( Fig. 2a , state I-b; ref. 37 ). While the tension was maintained, a mixture of staple strands, each strand at a concentration of 200 nM, was injected. Introduction of this staple-strand mixture induced further stretching of the scaffold DNA over 13±5 s ( n =18, Supplementary Fig. 3 ), indicating that the presence of the staple strands facilitated removal of residual internal structures ( Fig. 2a , state I-c). Under the 5 pN tension, the extension value culminated in a steady state. Significantly, the extension distribution of this steady state is very similar to that of the fully stretched scaffold DNA in its double-stranded form ( Fig. 2b ), implying that the state II that we anticipated above is obtained. 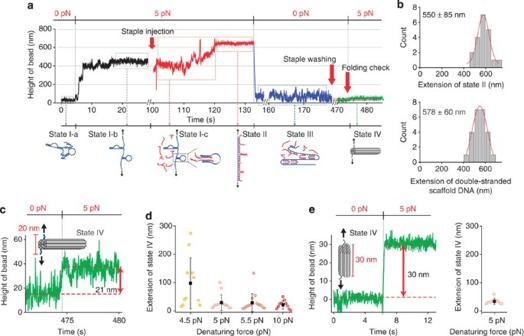Figure 2: Real-time observation of DNA nanostructure folding using magnetic tweezers. (a) Representative real-time extension trace of a single scaffold DNA during the folding process. Initially, the scaffold DNA has a compact secondary structure and its extension is almost zero (state I-a). Applying 5 pN to the scaffold DNA results in partial unfolding of the secondary structure (state I-b). Binding of staple strands further unfolds the internal structure of scaffold DNA (state I-c). When binding is finished, the scaffold DNA is in state II. Following magnetic force, quenching triggers strand displacement reactions among redundant staple strands (state III). After 5 min of folding at zero force, DNA nanostructure folding is checked by applying 5 pN of force (state IV). (b) The extension of state II (upper,n=24) and the extension of scaffold DNA in its double-stranded form (lower,n=20). The extension values were taken at 5 pN of force. Centre and width of distribution from Gaussian fits are 550±85 and 578±60 nm respectively. (c) Sample trace for the extension of DNA nanostructure. The extension was 21 nm, the expected change in distance for a correctly folded DNA nanostructure (Supplementary Fig. 7). (d) The extension of DNA nanostructures depending on the applied denaturing force. The average extension was significantly large for 4.5 pN of denaturing force (n=11, mean±s.d.=97±90 nm) than higher denaturing force, suggesting that at least 5 pN of force (n=13, mean±s.d.=30±27 nm) is required for proper folding (for 5.5 pN,n=13, mean±s.d.=28±31 nm; for 10 pN,n=10, mean±s.d.=21±15 nm). The data points are arranged in a manner that the largest extension value is placed at the centre and other data points are arranged in descending order in both directions. (e) The example trace for thick DNA nanostructure after folding (left). Collection of extensions are shown at the right side (n=9, mean±s.d.=34±10 nm). The data points are arranged in the same way as ind. Figure 2: Real-time observation of DNA nanostructure folding using magnetic tweezers. ( a ) Representative real-time extension trace of a single scaffold DNA during the folding process. Initially, the scaffold DNA has a compact secondary structure and its extension is almost zero (state I-a). Applying 5 pN to the scaffold DNA results in partial unfolding of the secondary structure (state I-b). Binding of staple strands further unfolds the internal structure of scaffold DNA (state I-c). When binding is finished, the scaffold DNA is in state II. Following magnetic force, quenching triggers strand displacement reactions among redundant staple strands (state III). After 5 min of folding at zero force, DNA nanostructure folding is checked by applying 5 pN of force (state IV). ( b ) The extension of state II (upper, n =24) and the extension of scaffold DNA in its double-stranded form (lower, n =20). The extension values were taken at 5 pN of force. Centre and width of distribution from Gaussian fits are 550±85 and 578±60 nm respectively. ( c ) Sample trace for the extension of DNA nanostructure. The extension was 21 nm, the expected change in distance for a correctly folded DNA nanostructure ( Supplementary Fig. 7 ). ( d ) The extension of DNA nanostructures depending on the applied denaturing force. The average extension was significantly large for 4.5 pN of denaturing force ( n =11, mean±s.d.=97±90 nm) than higher denaturing force, suggesting that at least 5 pN of force ( n =13, mean±s.d.=30±27 nm) is required for proper folding (for 5.5 pN, n =13, mean±s.d.=28±31 nm; for 10 pN, n =10, mean±s.d.=21±15 nm). The data points are arranged in a manner that the largest extension value is placed at the centre and other data points are arranged in descending order in both directions. ( e ) The example trace for thick DNA nanostructure after folding (left). Collection of extensions are shown at the right side ( n =9, mean±s.d.=34±10 nm). The data points are arranged in the same way as in d . Full size image Displacement among the staple strands was initiated by removing the magnetic force ( Fig. 2a , state III). Once a staple strand is removed from the scaffold DNA, it is unlikely to rebind because the local concentration of free staple strands is orders of magnitude lower than that of the bound staple strands ( Supplementary Fig. 4 ), implying that the displacement process is essentially irreversible. Fluctuation of the magnetic beads in lateral and vertical dimensions during the zero-force incubation step [38] shows that the folding process has been completed within 5 min ( Supplementary Fig. 5 ). We then washed away free staple strands through buffer exchange and raised the magnetic force back to 5 pN ( Supplementary Fig. 6 ). Remarkably, the extension of the scaffold DNA was dramatically reduced to 18±5 nm ( Fig. 2a,c,d ; state IV), an extension expected for the designed DNA nanostructure ( Supplementary Fig. 7 ). This observation suggests that the mechanical folding pathway has successfully folded the designed DNA nanostructure. It is worth noting that the entire folding process is completed within 8 min. We noticed that our folding protocol would work well with arbitrary force levels as long as the mechanical tension is large enough to successfully stretch the scaffold DNA. To explore this idea, we repeated our mechanical folding experiments while varying the denaturing force. As we observed that mechanical unfolding of our scaffold DNA requires at least 4.5 pN tension ( Supplementary Fig. 8 ), we first tried a denaturing force level of 4.5 pN, which is exactly the threshold force value and probably less efficient for inducing mechanical melting of the scaffold DNA. Indeed, this small difference in the denaturing force, as small as 0.5 pN, resulted in a much increased number of failure in the folding attempts as signified by the final extension values larger than 100 nm observed for the state IV ( Fig. 2d ). On the other hand, when the denaturing force is increased to 5.5 pN and to 10 pN, the final extension values of the state IV showed narrow distributions around 21 nm, indicative of formation of the desired DNA nanostructures. Finally, we wondered whether our folding pathway can be applied to different DNA nanostructures. We designed a honeycomb lattice of 19 helices with the same scaffold DNA ( Supplementary Fig. 9 and Supplementary Table 2 ). The folding protocol described in Fig. 2a was used with denaturing force of 5 pN. The extension values of the state IV showed a narrow distribution around 30 nm, which exactly matches with the expected value of 30 nm, that is, the distance between the two sides of the designed structure ( Fig. 2e ). We noticed that the number of helices in this structure is odd. Thus, the two DNA handles are attached to the opposite sides of the structure, respectively, unlike the previous case where the DNA handles are on the same side of the structure. Our observations indicate that this different geometry (that is, different way of scaffold-strand routing) does not hamper the folding process, suggesting that the mechanical folding protocol described here may be applicable to a range of different DNA nanostructures. Parallel folding of DNA origami with magnetic tweezers Next, we demonstrate that although our force control is at the single-molecule level, our folding scheme can fold multiple DNA nanostructures in a parallel manner. Among the tools for single-molecule force spectroscopy, magnetic tweezers uniquely permits parallel manipulation of many single molecules [31] , [35] , because the gradient of magnetic field is largely constant over a long length scale, for example, a millimetre scale for our magnet configuration [33] ( Supplementary Fig. 10 ). This suggests that when there are many scaffold DNAs in one force-acting area, the scaffold DNAs should fold into nanostructures at the same time after one force cycle ( Fig. 3 ). 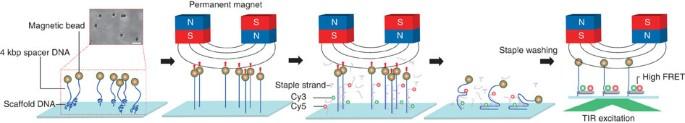Figure 3: Schematic for parallel DNA nanostructure folding with magnetic tweezers. Parallel force manipulation with magnetic tweezers folds many scaffold strands into DNA nanostructures in a single folding cycle. The left inset image shows example image of many magnetic beads immobilized in one imaging area. To check the folding with highly parallel manner, two staple strands were labelled with FRET pair Cy3 and Cy5 so that they show high FRET signal only after folding of DNA nanostructures. Single-molecule FRET signal was collected using TIR microscope. Figure 3: Schematic for parallel DNA nanostructure folding with magnetic tweezers. Parallel force manipulation with magnetic tweezers folds many scaffold strands into DNA nanostructures in a single folding cycle. The left inset image shows example image of many magnetic beads immobilized in one imaging area. To check the folding with highly parallel manner, two staple strands were labelled with FRET pair Cy3 and Cy5 so that they show high FRET signal only after folding of DNA nanostructures. Single-molecule FRET signal was collected using TIR microscope. Full size image To assess the folding of DNA nanostructures, we combined magnetic tweezers with a total internal reflection (TIR) microscopy that has detection sensitivity up to single-molecule fluorescence signals ( Fig. 3 and Supplementary Fig. 11 ; refs 21 , 34 ). We used the same design of DNA nanostructure, the honeycomb lattice of ten helices shown in Fig. 1b , with one difference that two of the staple strands were respectively labelled with Cy3 and Cy5 cyanine fluorophores, which constitute a dye pair for the single-molecule fluorescence resonance energy transfer (FRET) technique [39] . In the fully stretched scaffold DNA, these two fluorescent dyes are separated by a large distance (200 bp, Supplementary Fig. 1 ); however, when the scaffold DNA folds into a hexagonal bundle of ten helices, they are brought into close proximity with a separation less than 2 nm ( Fig. 3 and Supplementary Fig. 1 ). Thus, correct folding of the DNA nanostructure will lead to a drastic increase of the FRET efficiency. This method, combined with the wide-field imaging capability of TIR microscopy, provides a convenient way to assess the parallel folding of multiple scaffold DNAs. We prepared four different pairs of the labelled staple strands that were chosen to probe the folding status of different parts of the DNA origami structure ( Fig. 4a ). We formed the DNA nanostructures through a thermal annealing process and immobilized them on the imaging surface. When observed with our TIR microscopy, the first FRET pair, reporting the folding status of the distal part, showed a narrow FRET distribution around 0.9 ( Fig. 4b , black distribution). In contrast, simple mixing of scaffold DNA with the staple strands at room temperature resulted in low FRET efficiency values around 0.1 ( Fig. 4b , grey distribution). The other three FRET pairs also showed the high FRET values only after the thermal annealing process ( Fig. 4b ), confirming the validity of single-molecule FRET signal as a measure of correct folding. 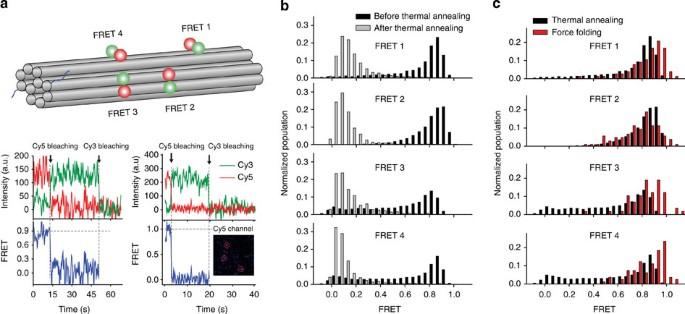Figure 4: Single-molecule FRET observation of parallel DNA nanostructure folding. (a) The position of four FRET pairs (upper). We labelled the rightmost pair as FRET pair 1. Representative single-molecule FRET traces of a DNA nanostructure folded with magnetic tweezers are shown (lower). Clear photobleaching steps of single donor and acceptor pair are observed. (b) Assessment of FRET efficiency. FRET efficiency of thermally annealed DNA nanostructures showed a high FRET peak (black distribution,n=1,927, 2,921, 830 and 1,222 for FRET 1, 2, 3 and 4, respectively), whereas simple mixing of staple strands with scaffold DNA showed a low FRET population (grey distribution,n=4,911, 9,442, 3,971 and 5,454 for FRET 1, 2, 3 and 4, respectively) for all 4 FRET pairs. (c) DNA nanostructures folded by magnetic tweezers give similar high FRET signal (red distribution,n=77, 106, 66 and 79 for FRET 1, 2, 3 and 4, respectively) to thermally annealed DNA nanostructures (black distribution), indicating successful nanostructure folding (Supplementary Fig. 14). Figure 4: Single-molecule FRET observation of parallel DNA nanostructure folding. ( a ) The position of four FRET pairs (upper). We labelled the rightmost pair as FRET pair 1. Representative single-molecule FRET traces of a DNA nanostructure folded with magnetic tweezers are shown (lower). Clear photobleaching steps of single donor and acceptor pair are observed. ( b ) Assessment of FRET efficiency. FRET efficiency of thermally annealed DNA nanostructures showed a high FRET peak (black distribution, n =1,927, 2,921, 830 and 1,222 for FRET 1, 2, 3 and 4, respectively), whereas simple mixing of staple strands with scaffold DNA showed a low FRET population (grey distribution, n =4,911, 9,442, 3,971 and 5,454 for FRET 1, 2, 3 and 4, respectively) for all 4 FRET pairs. ( c ) DNA nanostructures folded by magnetic tweezers give similar high FRET signal (red distribution, n =77, 106, 66 and 79 for FRET 1, 2, 3 and 4, respectively) to thermally annealed DNA nanostructures (black distribution), indicating successful nanostructure folding ( Supplementary Fig. 14 ). Full size image Using the parallel folding scheme described so far, we induced folding of many scaffold DNAs in one folding cycle and measured their FRET efficiencies. We immobilized about 30 scaffold DNAs in an area of 150 × 150 μm 2 and stretched them simultaneously by applying a magnetic force. To reduce autofluorescence from magnetic beads, we introduced a 4-kbp double-stranded DNA as a spacer between the magnetic bead and DNA nanostructure, which positioned the magnetic beads away from the evanescent excitation range of the TIR microscope ( Fig. 3 ). Staple strands were added to the reaction chamber for 1 min and the magnetic force was subsequently removed by moving the magnets away from the chamber, which completed one folding cycle after 5 min ( Fig. 3 ). Of note, the resulting DNA nanostructures on the imaging surface showed high FRET distributions for all the four FRET pairs ( Fig. 4c , red distributions) overlapping well with those of the thermally folded DNA nanostructures ( Fig. 4c , red versus black distributions). We checked the photobleaching of dyes to ensure that the signal from a nanostructure originated from single-molecule FRET ( Fig. 4a and Supplementary Fig. 12 ). Finally, mechanical stretching with very high force (tens of pN) reveals that our force-induced DNA nanostructure has a mechanical stability comparable to that of the thermally folded structures ( Supplementary Fig. 13 ). These findings indicate that our folding protocol using magnetic tweezers promotes correct and rapid folding of DNA nanostructures in a parallel manner. We compare the two folding pathways for DNA nanostructures, thermal and mechanical folding pathways, through illustration of each process in the folding landscape [27] . In the thermal folding protocol, the scaffold DNA, initially trapped in one of its secondary structures, is first brought to the thermally denatured ensembles with high entropy ( Fig. 5 , black arrow). Through a subsequent cooling step, the scaffold DNA and staple strands are slowly annealed into the designed nanostructure ( Fig. 5 , black arrow). A complicated, disordered mixture of molecular processes occurs during the thermal annealing, which includes binding and displacement of staple strands and refolding of the scaffold DNA into secondary structures. The landscape of thermal folding is rugged in part because of recurring secondary structures in the scaffold DNA. 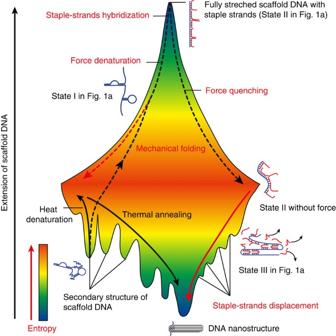Figure 5: Illustration of two different folding pathways of DNA nanostructure. In the conventional folding protocol using temperature control, the scaffold DNA is located at one of its secondary structures. During thermal folding cycle, the scaffold DNA is denatured at a high-temperature step (black arrow) and then slowly annealed to designed DNA nanostructure through rugged folding landscape (black arrow). Using magnetic tweezers, the scaffold DNA is stretched to the force-denatured state by 5 pN of force (black dashed arrow). Without staple strand binding, the scaffold DNA is refolded into one of its self-fold states on force quench (red dashed arrow). On staple strand binding (state II), the scaffold DNA follows a different pathway on force quench (black dashed arrow), because secondary structure is prevented. Along the folding pathway generated by the force-quench protocol (red arrow), the scaffold DNA folds to the designed nanostructure by overcoming small barriers associated with each strand-displacement reaction in which a redundant staple strand is released from the scaffold DNA. Figure 5: Illustration of two different folding pathways of DNA nanostructure. In the conventional folding protocol using temperature control, the scaffold DNA is located at one of its secondary structures. During thermal folding cycle, the scaffold DNA is denatured at a high-temperature step (black arrow) and then slowly annealed to designed DNA nanostructure through rugged folding landscape (black arrow). Using magnetic tweezers, the scaffold DNA is stretched to the force-denatured state by 5 pN of force (black dashed arrow). Without staple strand binding, the scaffold DNA is refolded into one of its self-fold states on force quench (red dashed arrow). On staple strand binding (state II), the scaffold DNA follows a different pathway on force quench (black dashed arrow), because secondary structure is prevented. Along the folding pathway generated by the force-quench protocol (red arrow), the scaffold DNA folds to the designed nanostructure by overcoming small barriers associated with each strand-displacement reaction in which a redundant staple strand is released from the scaffold DNA. Full size image In our mechanical folding protocol, the scaffold DNA goes through microstates that would be very improbable to visit in a thermally driven process. First, the scaffold DNA is stretched to a force-denatured ensemble with low entropy ( Fig. 5 , black dashed arrow). Without staple strands, the scaffold DNA would return to one of its secondary structures when the mechanical tension is removed ( Fig. 5 , red dashed arrow). Hybridization with staple strands, however, drives the scaffold DNA to a totally different state (that is, State II without force in Fig. 5 ), while inhibiting formation of secondary structures. In the final step of our mechanical folding pathway, there are energetic barriers presented by the displacement reaction of the bound staple strands ( Fig. 5 , red arrow). We notice that these barriers for the displacement reaction are much smaller in magnitude than those for opening secondary structures of the scaffold DNA, which makes our folding pathway smooth and efficient in speed. Our mechanical folding pathway consists of an ordered and well-separated sequence of three molecular processes: stretching of the scaffold DNA, staple-strands binding and displacement between the redundant staple strands. As the three molecular processes are simple and well characterized, the time required to complete a folding cycle can be quantitatively predicted. The first step, mechanical unfolding of the scaffold DNA, usually takes <10 s ( Fig. 2a ). The second process, hybridization of staple strands with the stretched scaffold DNA is essentially the same as solid-phase oligo hybridization [40] , and should thus be completed within 1 min when each staple strand is present at 200 nM. Time required for the strand displacement reaction depends on the number of strands to be displaced and the length of binding sites [30] . We presume that the ten helices in our honeycomb lattice undergo folding in a parallel manner. Ten displacement reactions with an average binding site of 8 bp are required to fold one helix in our DNA origami design, which takes about 5 min at room temperature [30] . For more accurate estimation, staple strand exchange should also be considered, because the existence of some staple strand exchange was observed ( Supplementary Fig. 6 ). As a result, the total time required for one folding cycle is estimated to be 7 min, which is close to the experimentally determined time of 8 min ( Fig. 2a ). This folding speed is comparable to the recently demonstrated constant-temperature incubation [16] . In our mechanical folding method, a small heterogeneity in force is tolerable as long as the force is large enough to stretch the scaffold DNAs. This also suggests that we can even fold different DNA nanostructures at the same time. This parallel folding, combined with automated large-scale force control (for example, using electromagnetic force or flow-induced Stokes force), may eventually enable mass production of DNA nanostructures. At the same time, our mechanical folding pathway may provide an avenue towards programmed assembly of DNA nanostructures. One possibility is part-by-part assembly, in which a DNA nanostructure with multiple parts can be sequentially folded in independent folding cycles, which use different sets of staple strands that constitute different parts of the DNA nanostructure. Preparation of scaffold strand A 1,898-bp fragment of λ -DNA (27,945–29,843, from New England Biolabs) was amplified by PCR using 5′-digoxigenin-modified antisense primer (all primers were purchased from Integrated DNA Technologies). Purified PCR products were digested with BamHI-HF (New England Biolabs) and ligated with short double-stranded DNA that had 3′-biotin. The antisense strand of the DNA was modified with 3′-biotin and 5′-digoxigenin. This double-stranded DNA was then attached to streptavidin-coated magnetic bead (Invitrogen), following a standard protocol provided by the manufacturer. Typically, 100 μl of 200 nM DNA solution was mixed with 400 μl of magnetic bead solution. After removing unbound DNA by taking the supernatant, the magnetic bead was further washed with distilled water twice. Next, we added 200 μl of 20 mM NaOH solution to the magnetic bead that denatures double-stranded DNA, removing the sense strand from the magnetic bead. Then, we washed the magnetic bead again with distilled water twice. The antisense strand was released from the bead by heating the sample to 63 °C in 200 μl of distilled water [41] . Typical concentration of resulting single-stranded DNA was 40 nM in 200 μl. Following this single-stranded DNA purification cycle, scaffold DNA was further concentrated ten times using DNA concentration kit (Oligo clean and concentrator, Zymoresearch) and stored at −20 °C for further use. DNA nanostructure design DNA nanostructures were designed using caDNAno with hexagonal geometry [42] . We introduced a short, 30-bp double-stranded linker region on the top and bottom of the DNA nanostructure (referred to as the upper and lower linker, respectively, in the main text), to reduce the effect of surface for folding process. Detailed structures including strand-routing diagram and position of fluorophore-modified staple strands can be found in Supplementary Figs . Sequence of staple strands are shown in Supplementary Tables . Staple strands were dissolved in distilled water at 100 μM and stored at −20 °C. Staple strand master mix for each structure, which contains 2 μM of each staple strand, was also prepared and stored for further use. Preparation of sample chamber for magnetic tweezers Sample chamber with PEG- and biotin-PEG-coated cover slide was prepared as previously described [26] . We first attached neutravidin to biotin-PEG by injecting 50 μl of 100 μg ml −1 of neutravidin solution in T50 buffer (10 mM Tris–HCl, 50 mM NaCl, pH 8.0) and incubating for 5 min. After washing out extra neutravidin with 200 μl of TE buffer (description) twice, 40 μl of 10 nM scaffold DNA solution was injected and incubated for 10 min. After washing out twice with 200 μl of PBST buffer (PBS supplemented with 0.1% of Tween 20), 40 μl of reference bead (streptavidin-coated polystyrene bead, 1-μm radius, Polyscience) dissolved in PBS was immobilized for 3 min. After washing out twice with 200 μl of PBST buffer, anti-digoxigenin (Roche)-coated magnetic bead (Dynabead, Invitrogen) with 1 or 2.8-μm diameter was attached to the digoxigenin-modified 5′-end of scaffold DNA by injecting 40 μl of magnetic bead solution. Magnetic bead with 2.8 μm diameter was used only when higher magnetic force was required (the 10-pN data points in Fig. 2d and Supplementary Fig. 13 ). After 30 min, we washed out extra magnetic bead with 200 μl of PBST buffer twice. Folding of DNA nanostructure using magnetic tweezers Home-built magnetic tweezers were constructed as described [26] . A pair of permanent magnets, vertically controlled by a translational motor (Physik Instrumente, M-126.PD1), was used to apply force to the magnetic beads. The magnetic beads were illuminated with a blue light-emitting diode over the magnets and the diffraction patterns of the beads were imaged by a charge-coupled device (CCD) camera (JAI, CM-040GE). The integrity of single-stranded DNA was assessed by applying 5 pN of force in PBST buffer. Only the molecules showing force extension of single-stranded DNA, including hairpin-like transition and characteristic extension (around 600 nm), were selected for further experiment. After changing buffer to folding buffer (12 mM MgCl 2 , 5 mM NaCl, 10 mM Tris–HCl, 1 mM EDTA, 0.1% Tween 20, 0.1 mg ml −1 of BSA, pH 8.0), we applied 5 pN of denaturing force to the scaffold DNA unless stated otherwise. We checked the integrity of scaffold DNA again in the folding buffer. While maintaining the denaturing force, we injected folding solution (200 nM of each staple strand dissolved in folding buffer) to the chamber. After the injection of staple strands, we waited 1 min to induce complete binding of staple strands. Next, the displacement reaction was initiated by moving magnets away from the sample slide. The position of magnetic bead was monitored during the displacement reaction. After 5 min of displacement reaction, we checked the folding of DNA nanostructures by applying 5 pN of force. All reaction was carried out at 36 °C using temperature controller for Olympus microscope (Live Cell Instrument). Thermal folding of DNA nanostructures We prepared 30–50 μl of reaction mixture that contains 20 nM of scaffold DNA, 200 nM of each staple strand in folding buffer (12 mM MgCl 2 , 5 mM NaCl, 10 mM Tris–HCl, 1 mM EDTA, pH 8.0). The reaction mixture was briefly heat denatured at 80 °C for 5 min and then slowly cooled from 80 °C to 60 °C at the rate of 1 °C per 15 min, and then cooled from 60 °C to 25 °C at the rate of 0.5 °C per 45 min in a thermal cycler (Applied Biosystems). Electron microscope imaging of thermally folded DNA nanostructures A 3-μl aliquot of DNA nanostructure (10 nM in 50 mM NaCl, 12 mM MgCl 2 ) was adsorbed onto negatively glow discharged (PELCO easiGlow) transmission electron microscope grids for 30 s. The grids were stained with 0.75% uranyl formate and imaged with a SC1000 CCD camera (Gatan Inc.) on JEM-3011HR (JEOL Ltd, Japan) operating at 300 kV. The magnification for the image was 50,000. Single-molecule FRET measurement For thermally folded DNA nanostructures, sample chamber using PEG-coated quartz slide was prepared as previously described [43] . TIR fluorescence microscope for Cy3-Cy5 FRET measurement is described elsewhere [44] . We injected 80 μl of 1–10 μg ml −1 of neutravidin (Invitrogen) solution into the chamber and waited for 5 min to prepare neutravidin-covered surface. During the incubation, thermally folded DNA nanostructures with biotin at the 3′-end was diluted to 10 μM in folding buffer. Free neutravidin in chamber was removed by washing with 400 μl of folding buffer. Next, 80 μl of the DNA nanostructure solution was injected and incubated for 5 min. The FRET efficiency of DNA nanostructure was measured using home-built TIR microscope in the presence of an imaging buffer system [45] . Hybrid setup that combines magnetic tweezers and objective-type TIR microscopy for single-molecule FRET measurement was used to confirm force-controlled origami folding, using single-molecule FRET ( Supplementary Fig. 9 ). The fluorescent dyes were illuminated by objective-type TIR. A green laser beam (532 nm, Thorlabs) was allowed to enter through the back port of the microscope, with beam splitters in the microscope (Semrock, Di02-R532-25 × 36 for 532 nm and Di02-R635-25 × 36 for 638 nm) reflecting the beams towards the imaging spot. The epi-fluorescence mode was switched to the TIR mode by shifting the beam path to the edge of the objective lens. The excitation beam and the Cy3/Cy5 emissions were passed through the beam splitters and excitation lasers were filtered by long-pass filters (Semrock, LP03-532RS-25 for 532 nm and LP02-633RS-25 for 638 nm). An emission splitter (Semrock, FF640-FDi01-25 × 36) was used to separate the Cy3 and Cy5 emissions. The background signal was further suppressed by a Cy3/Cy5 dual-band bandpass filter (Semrock, FF01-577/690-25) in front of the electron-multiplying CCD. As magnetic beads showed significant autofluorescence in green, we added 4,000-bp double-stranded DNA (contour length, 1,360 nm) to the upper end of the scaffold strand to place the magnetic beads away from the evanescence field excitation region (~300 nm from the surface). This spacer DNA was restricted by BamHI (New England Biolabs) and then ligated with single-stranded scaffold DNA using Taq DNA ligase (New England Biolabs). Next, this combined single-stranded scaffold strand and double-stranded spacer DNA were similarly incubated, immobilized and folded into DNA nanostructures using the same folding protocol. After folding, remaining staple strands were removed by washing with 200 μl of folding buffer. The FRET efficiency was measured in the presence of imaging buffer [45] , with 4 pN of magnetic force to reduce the autofluorescence from magnetic beads. Only the molecules that showed clear photobleaching in a single step were selected for analysis. How to cite this article : Bae, W. et al . Programmed folding of DNA origami structures through single-molecule force control. Nat. Commun. 5:5654 doi: 10.1038/ncomms6654 (2014).